Catalytic site remodelling of the DOT1L methyltransferase by selective inhibitors Selective inhibition of protein methyltransferases is a promising new approach to drug discovery. An attractive strategy towards this goal is the development of compounds that selectively inhibit binding of the cofactor, S -adenosylmethionine, within specific protein methyltransferases. Here we report the three-dimensional structure of the protein methyltransferase DOT1L bound to EPZ004777 , the first S -adenosylmethionine-competitive inhibitor of a protein methyltransferase with in vivo efficacy. This structure and those of four new analogues reveal remodelling of the catalytic site. EPZ004777 and a brominated analogue, SGC0946 , inhibit DOT1L in vitro and selectively kill mixed lineage leukaemia cells, in which DOT1L is aberrantly localized via interaction with an oncogenic MLL fusion protein. These data provide important new insight into mechanisms of cell-active S -adenosylmethionine-competitive protein methyltransferase inhibitors, and establish a foundation for the further development of drug-like inhibitors of DOT1L for cancer therapy. Protein methyltransferases (PMTs) have essential roles in epigenetic regulation of gene expression and chromatin-dependent signalling via their methylation of histones and other chromatin-associated substrates. Mutation or misregulation of PMTs is linked to many diseases, especially cancer, and there is strong interest in this family of proteins as potential drug targets [1] , [2] , [3] . Targeting the common S -adenosylmethionine (SAM) cofactor-binding site of PMTs is an attractive strategy for this family, analogous to targeting the ATP-binding site of protein kinases [4] , [5] . There are 60 PMTs encoded in the human genome, including 51 lysine methyltransferases (PKMTs) and 9 protein arginine methyltransferases (PRMTs) [1] . Most PKMTs contain a conserved SET domain, with the exception of DOT1L, which has a protein fold that more closely resembles PRMTs [6] . DOT1L is also unique in that it is the only PKMT to methylate histone H3 on Lysine 79 (H3K79) [7] , [8] , a chromatin mark associated with active chromatin and transcriptional elongation [9] . Aberrant mono- and dimethylation of H3K79 by DOT1L is an essential step in the development of MLL-rearranged mixed lineage leukaemia, an acute form of the disease that, in infants, constitutes 70% of acute lymphoid and over 35% of acute myeloid leukemias [10] , [11] , [12] , [13] . MLL-rearranged mixed lineage leukaemia is driven by chromosomal translocations that result in an oncogenic fusion protein comprising the amino terminal region of MLL and the carboxy terminus of one of ~70 translocation partners [14] , and pharmacological targeting of MLL translocation complexes was recently shown to reverse oncogenic activity of MLL fusion proteins in leukemia [15] . A subset of MLL fusion partners, including AF4, AF9 and AF10, aberrantly recruit DOT1L to select genomic loci leading to increased H3K79 methylation and transcriptional activation of genes essential for leukemogenesis [16] . Recently, the antileukemic activity of DOT1L inhibition by either genetic or pharmacological approaches resulted in selective killing of MLL-AF4/9/10 translocation carrying cells [10] , [17] . In particular, EPZ004777 ( Fig. 1c ), a picomolar, specific, SAM-competitive inhibitor of DOT1L, selectively kills cells bearing MLL chromosomal rearrangements and extends survival in a murine xenograft model of MLL [17] . DOT1L inhibition by EPZ004777 also accelerated reprogramming of somatic cells into induced pluripotent stem cells [18] , suggesting that DOT1L inhibition may be useful in regenerative medicine. 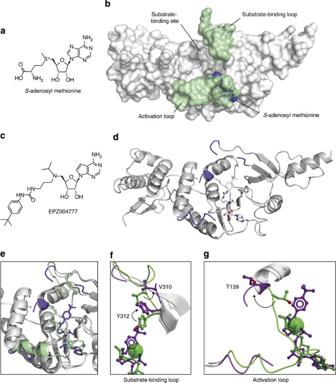Figure 1: Structural mechanism of DOT1L inhibition. Binding of the cofactor SAM (a) stabilizes a catalytically competent conformation of DOT1L where the activation and substrate-binding loops (green) guide the substrate towards the site of methyl transfer (b). Binding ofEPZ004777(c) affects the conformation of these loops, which become partly disordered (d-magenta).EPZ004777occupies the same site as SAM (e), but conformational rearrangement of substrate-binding and activation loop residues (f,g, respectively) are necessary to accommodate the t-butylphenyl group. Figure 1: Structural mechanism of DOT1L inhibition. Binding of the cofactor SAM ( a ) stabilizes a catalytically competent conformation of DOT1L where the activation and substrate-binding loops (green) guide the substrate towards the site of methyl transfer ( b ). Binding of EPZ004777 ( c ) affects the conformation of these loops, which become partly disordered ( d -magenta). EPZ004777 occupies the same site as SAM ( e ), but conformational rearrangement of substrate-binding and activation loop residues ( f , g , respectively) are necessary to accommodate the t-butylphenyl group. Full size image To understand the structural mechanism of SAM-competitive inhibition of PMTs, and of DOT1L in particular, we solved the structure of DOT1L in complex with EPZ004777 , and uncovered novel and unexpected conformational variability of the cofactor-binding site that can accommodate compounds significantly larger and more hydrophobic than SAM. We also present chemical analogues with improved solubility or potency including SGC0946 , a compound significantly more potent than EPZ004777 in cells, which will serve as a useful chemical probe of DOT1L [19] . These results provide important insight into SAM-competitive inhibition of HMTs in general, and reconcile the contradictory observations that both very polar and very hydrophobic compounds can bind at the DOT1L cofactor site. Our data will also guide the design of new inhibitors with improved drug-like properties. Conformational rearrangement of DOT1L by EPZ004777 The catalytic subunit of DOT1L comprises its first 416 residues [6] . Mono- and dimethylation of H3K79 is dependent on SAM ( Fig. 1a ), which binds within a cofactor-binding site that is largely enclosed by an activation loop (residues 122–140; Fig. 1b ). Structural and biochemical studies by Rui-Ming Xu and colleagues characterize a 4-Å methyl transfer channel partitioning the SAM-binding cavity from the putative substrate-binding site, which is formed by a substrate-binding loop (residues 301–311). This spatial organization is consistent with an in-line methyl transfer reaction, whereby a likely deprotonated acceptor lysine executes nucleophilic attack on the SAM methyl group [6] . EPZ004777 ( Fig. 1c ) is a near chemical derivative of SAM that inhibits DOT1L with extraordinary potency in a radionuclide homogeneous assay (IC 50 =400 pM), and possesses surprising selectivity for DOT1L compared with other SAM-dependent lysine and arginine methyltransferases [17] . Limited information is available regarding the design of EPZ004777 , but most striking is the para-tert-butylphenyl appending group coupled via a urea linkage. Structural modelling studies of EPZ004777 bound to the SAM-binding pocket of DOT1L [PDB:1NW3] failed to identify a ligand conformation that could accommodate this bulky substituent within the enclosed amino-acid-binding pocket. The only pose of EPZ004777 with a suitable fit within the DOT1L active site was accomplished by telescoping the urea capping feature through the methyl transfer channel and into the substrate-binding site (data not shown). To resolve the binding mechanism definitively, we crystallized a complex of DOT1L bound to EPZ004777 by soaking a crystal of DOT1L in complex with the reaction by-product S -adenosylhomocysteine (SAH) in a solution of EPZ004777 . The binary crystal structure of DOT1L in complex with EPZ004777 was solved to a resolution of 2.4 Å (PDB code 4ER3; Supplementary Table S1 , Supplementary Figs S1, S2 ). The overall structure is very similar to that of DOT1L bound to SAM (1.1 Å backbone RMSD relative to PDB code 1NW3) with the exception of the activation and substrate-binding loops, which are disordered in the EPZ004777 -bound structure ( Fig. 1d ). As expected, EPZ004777 occupies the cofactor-binding site, and, consistent with molecular modelling, the t-butylphenyl moiety of EPZ004777 cannot fit in the SAM-bound conformation of the cofactor pocket. Large structural rearrangements at Tyr312 and Thr139, in the substrate-binding and activation loops, respectively, are necessary to accommodate this portion of the inhibitor ( Fig. 1f–g ). Importantly, Tyr312 and Thr139 are considered key partners in forming the methyl transfer channel, and mutation of Tyr312 to Ala abrogates methyltransferase activity [6] . In the presence of EPZ004777 , Tyr312 is rotated away from this channel to accommodate the t-butyl moiety ( Fig. 1f ) while Thr139 is repositioned ~6 Å away from its SAM-bound state ( Fig. 1g ). These conformational changes therefore disrupt the structural integrity of the catalytic pocket, and must necessarily propagate along the activation and substrate-binding loops, possibly further disrupting these catalytically important structural features ( Fig. 1e ). Unexpectedly, EPZ004777 adopts an extended conformation in the complex structure, and multiple interactions scattered along the inhibitor likely contribute to its potent binding. The deazaadenosine moiety of the inhibitor recapitulates critical interactions with Glu186, Asp222 and Phe223 previously observed with SAM, SAH and close cofactor mimetics ( Fig. 2a ) [5] , [6] , [20] . The t-butylphenyl end of the compound is surrounded by a cluster of hydrophobic sidechains (L143, V144, M147, V169, F239, V267 and Y312). The urea linker is elegantly exploited via interaction with the carboxylic group of D161, and the protonated nitrogen of the isopropyl ammonium is favourably engaged in a hydrogen bond with the backbone carbonyl of G163. However, it is not clear whether the hydrophobic isopropyl moiety is interacting favourably with the activation loop, which is disordered in our structure. Finally, a hydrophobic cleft composed of sidechains from F223, F245 and V249 located in close proximity to position 7 of the deazaadenine ring remains unexploited ( Fig. 2b ). 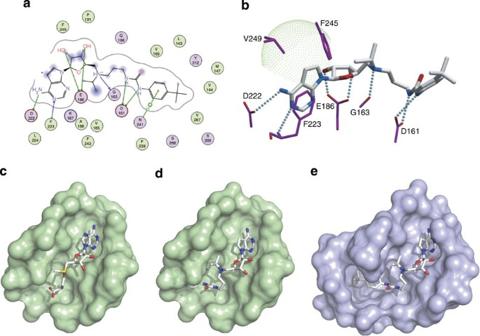Figure 2: Molecular recognition of the DOT1L cofactor pocket byEPZ004777 (a) Two-dimensional projection of DOT1L–EPZ004777interactions generated with MOE (Chemical Computing Group, Montreal, Canada). Residues within 4.5 Å of the ligand are shown, unless they form no hydrogen bond and their sidechains are pointing away from the inhibitor. Grey line: DOT1L surface envelope; blue shading: solvent accessibility; hydrogen bonds with DOT1L sidechain/backbone atoms: green/blue arrows; green aromatic rings symbolize arene-cation interactions; amino-acid colour code is pink: polar, green: hydrophobic, blue rim: basic, red rim: acidic. Position 7 ofEPZ004777is indicated by a star. (b) Three-dimensional representation highlighting hydrogen bonds that mediate the interaction (doted lines) and a hydrophobic cluster (green sphere) that is not exploited byEPZ004777. (c) Cofactor-binding site in complex with SAM (PDB code 1NW3). (d) The t-butylphenyl group ofEPZ004777does not fit in the SAM-bound conformation of DOT1L. (e) Conformational rearrangements of DOT1L open up a cavity to accommodate the t-butylphenyl group. Figure 2: Molecular recognition of the DOT1L cofactor pocket by EPZ004777 ( a ) Two-dimensional projection of DOT1L– EPZ004777 interactions generated with MOE (Chemical Computing Group, Montreal, Canada). Residues within 4.5 Å of the ligand are shown, unless they form no hydrogen bond and their sidechains are pointing away from the inhibitor. Grey line: DOT1L surface envelope; blue shading: solvent accessibility; hydrogen bonds with DOT1L sidechain/backbone atoms: green/blue arrows; green aromatic rings symbolize arene-cation interactions; amino-acid colour code is pink: polar, green: hydrophobic, blue rim: basic, red rim: acidic. Position 7 of EPZ004777 is indicated by a star. ( b ) Three-dimensional representation highlighting hydrogen bonds that mediate the interaction (doted lines) and a hydrophobic cluster (green sphere) that is not exploited by EPZ004777 . ( c ) Cofactor-binding site in complex with SAM (PDB code 1NW3). ( d ) The t-butylphenyl group of EPZ004777 does not fit in the SAM-bound conformation of DOT1L. ( e ) Conformational rearrangements of DOT1L open up a cavity to accommodate the t-butylphenyl group. Full size image Overall, comparison of DOT1L bound to SAM (1NW3) and EPZ004777 (4ER3) reveals structural remodelling of the catalytic site ( Fig. 2c–e ). SAM exhibits excellent shape complementarity with the internal face of the binding pocket ( Fig. 2c ), whereas EPZ004777 is incompatible with this pocket geometry ( Fig. 2d ). Visualization of the internal face of the SAM-binding pocket in the EPZ004777 complex reveals a new internal cavity formed around the t-butylphenyl feature ( Fig. 2e ). Thus, our structure clearly indicates positions—such as the urea and t-butylphenyl group—that make favourable interactions, and other positions—such as the deazaadenosine moiety—that can be further explored to improve potency. Structure-guided exploration of key inhibitory features To explore putative determinants of molecular recognition, we prepared a focused library of analogous molecules to EPZ004777 for biochemical and biophysical study ( Table 1 ), using an efficient seven-step synthesis ( Supplementary Methods ). Taking advantage of the hydrophobic cleft in DOT1L surrounding position 7 of the adenine ring, we synthesized SGC0946 , an EPZ004777 analogue with a bromine atom at position 7, which is expected to increase potency by occupying this cleft. Indeed, SGC0946 is a more potent DOT1L inhibitor than EPZ004777 . Surface plasmon resonance (SPR) and a homogeneous biochemical assay with recombinant, purified DOT1L acting on a nucleosomal substrate yielded a K D of 0.25±0.02 nM and IC 50 of 0.5±0.1 nM for EPZ004777 (in agreement with previous work [17] ), while a K D of 0.06 nM and IC 50 0.3±0.1 nM were measured for SGC0946 ( Table 1 ; Fig. 3a ). The gain in potency was even more substantial in cells: the brominated compound reduced the level of methylation of H3K79 in MCF10A cells with an IC 50 of 8.8±1.6 nM, compared with an IC 50 of 84±20 nM for EPZ004777 , as measured by whole-cell immunofluorescence (in-cell western assay) ( Fig. 3d ). Bromination of the adenine ring did not affect selectivity: like EPZ004777 , SGC0946 was inactive against a panel of 12 PMTs and DNMT1 ( Supplementary Fig. S3 ). We found both compounds inactive against PRMT5, while an IC 50 of ~500 nM was originally reported for EPZ004777 [17] . This discrepancy may come from the fact that our assay is based on the PRMT5–MEP50 complex, while the previously reported inhibition was for isolated PRMT5. Table 1 Biochemical and cellular assay summary of EPZ004777 and analogues. 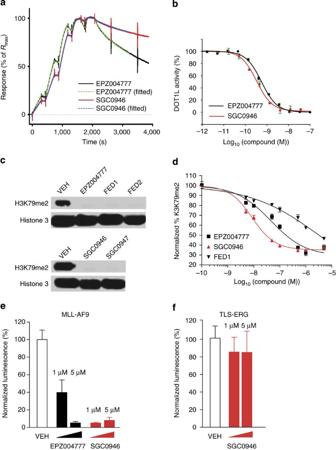Figure 3: Biochemical and cellular characterization of DOT1L inhibitors. (a) Biacore SPR sensorgram from single-cycle kinetics runs with five concentrations, normalized to the calculated Rmax, indicate thatEPZ004777andSGC0946bind to DOT1L with 1:1 stoichiometry and dissociation constants (KD) of 0.25 and 0.06 nM, respectively. (b)EPZ004777andSGC0946inhibit DOT1L enzymatic activity with IC50values of 0.5 and 0.3 nM, respectively. (c) Inhibition of H3K79me2 by a series of DOT1L inhibitors measured by immunoblot (10 μM exceptSGC0946, 1 μM; 4 days) and (d) cellular H3K79 methylation assay using fluorescence microscopy. (e)SGC0946(1 and 5 μM) kills human cord blood cells transformed with an MLL–AF9 fusion oncogene, whileEPZ004777was less efficacious at the lower concentration (1 μM). (f)SGC0946(1 and 5 μM) does not affect viability of cord blood cells transformed with an unrelated oncogene, TLS-ERG. VEH: DMSO control. Error bars represent s.e. of the mean from at least two independent experiments, with each experiment representing three repeats. Full size table Figure 3: Biochemical and cellular characterization of DOT1L inhibitors. ( a ) Biacore SPR sensorgram from single-cycle kinetics runs with five concentrations, normalized to the calculated Rmax, indicate that EPZ004777 and SGC0946 bind to DOT1L with 1:1 stoichiometry and dissociation constants ( K D ) of 0.25 and 0.06 nM, respectively. ( b ) EPZ004777 and SGC0946 inhibit DOT1L enzymatic activity with IC 50 values of 0.5 and 0.3 nM, respectively. ( c ) Inhibition of H3K79me2 by a series of DOT1L inhibitors measured by immunoblot (10 μM except SGC0946 , 1 μM; 4 days) and ( d ) cellular H3K79 methylation assay using fluorescence microscopy. ( e ) SGC0946 (1 and 5 μM) kills human cord blood cells transformed with an MLL–AF9 fusion oncogene, while EPZ004777 was less efficacious at the lower concentration (1 μM). ( f ) SGC0946 (1 and 5 μM) does not affect viability of cord blood cells transformed with an unrelated oncogene, TLS-ERG. VEH: DMSO control. Error bars represent s.e. of the mean from at least two independent experiments, with each experiment representing three repeats. Full size image Structural advantages to the position 7 substitution of the basic adenine nitrogen with carbon in EPZ004777 were not identified. Indeed, this modification serves to impair solubility and increase the complexity and expense of the synthetic effort. We therefore prepared the adenine derivative, FED1 , which demonstrates potent inhibitory activity for DOT1L in homogeneous (IC 50 =2.9±0.2 nM) and cell-based (IC 50 =1.4 μM) assays ( Table 1 , Fig. 3d ). To confirm that the hydrophobic interactions at the t-butyl group of EPZ004777 contribute significantly to binding, we synthesized FED2 , a derivative of FED1 in which the t-butyl was replaced by a methyl group. FED2 exhibited a reduction in target potency in biochemical (IC 50 =40.3±7.3 nM) and biophysical ( K D =26.9 nM) assays. We also investigated the importance of the isopropyl group by measuring the effect of its deletion from SGC0946 . The resulting compound ( SGC0947 ) had a tenfold increase in IC 50 , which reflects a non-negligible contribution of this group to the interaction. Finally, we verified with the EPZ004777 analogue EJC1 that replacing the essential urea linker by an amide bond abrogated inhibitory activity. We next tested the active compounds, EPZ004777 , FED1 , FED2 , SGC0946 and SGC0947 , in several MLL and non-MLL cell lines in order to assess their effects on DOT1L cellular function. Depletion of H3K79me2 was evident at 48 h for all compounds in MV4;11 leukaemia cells expressing an MLL/AF4 fusion protein ( Fig. 3c ). Similarly, EPZ004777 and SGC0946 both showed time- and dose-dependent reductions in the H3K79me2 mark in the Molm13 MLL cell line that has the MLL/AF9 translocation ( Supplementary Fig. S4a ). Quantitative assessment of H3K79me2 levels as measured by automated epifluorescence microscopy in MCF10A cells ( Table 1 , Fig. 3d ) showed a substantially improved DOT1L inhibitory potency of SGC0946 (IC 50 =8.8±1.6 nM) compared with EPZ004777 (IC 50 =84±20 nM). A similar observation was made in A431 cells, with IC 50s of 2.65 nM and 264 nM for SGC0946 and EPZ004777 , respectively ( Supplementary Fig. S4b ). We attribute this increase in cellular potency to lower off-rate as measured by SPR experiments, which results in extended residence time of SGC0946 ( K off =1.5E–4 s −1 ) compared with EPZ004777 ( K off =9.29E–4 s −1 ) ( Fig. 3a ; Supplementary Fig. S5 ) [21] , and to improved apparent permeability ( Supplementary Table S2 ). Consistent with a biologically selective effect on DOT1L, SGC0946 displayed selective reduction of cell viability in an experimental leukaemia model derived from human cord blood cells transformed with the MLL-AF9 fusion oncogene [22] , without apparent effect on the viability of cells transformed with an MLL-unrelated translocation (TLS-ERG) [23] ( Fig. 3e ). SGC0946 also showed increased efficacy in this model relative to EPZ004777 . In addition, SGC0946 at 1 μM effectively lowered the levels of MLL target genes, HOXA9 and Meis1 ( Supplementary Fig. S4c,d ). Chances that cellular activity of SGC0946 is mediated by off-target effect are low considering its lack of activity against a panel of 29 diverse receptors ( Supplementary Table S3 ). Taken together, these data demonstrate a consistent trend between in vitro biochemical and biophysical activity, and selective, on-target cellular activity of DOT1L inhibitors. Two loops at the catalytic site adopt multiple conformations To verify that the binding mode of EPZ004777 is conserved with that of its chemical analogues, the DOT1L structure was solved in complex with the four active derivatives. As expected, the compounds recapitulated the EPZ004777 -binding pose ( Fig. 4a Supplementary Figs S1, S2 ). Strikingly, however, each of the four structures captured the activation and substrate-binding loops in a different conformation. The activation loop was fully ordered only in the DOT1L– FED2 complex while the substrate-binding loop was ordered in all four complex structures ( Fig. 4a ). The lack of completeness of the electron density at the activation loop in some structures may reflect a partial occupation of the cofactor site by inhibitors ( Supplementary Fig. S2 ). While the original DOT1L– EPZ004777 structure was obtained by soaking a crystal of the DOT1L–SAH complex in a solution of EPZ004777 , this new series of structures was produced by soaking crystals of DOT1L in complex with 5-iodotubercidin, a kinase inhibitor that we had previously identified as weakly inhibiting DOT1L (IC 50 =18±0.9 μM; Supplementary Fig. S3 ). Unlike the crystals of the DOT1L–SAH complex, which generally broke during soaking and rarely allowed displacement of SAH by the inhibitors, we found soaking experiments much more efficient with the DOT1L–5-iodotubercidin crystals. Surprisingly, when we soaked the latter in a solution of EPZ004777 , we found two molecules of EPZ004777 bound to a single DOT1L molecule. One EPZ004777 ligand was in the SAH-binding pocket, in the same pose as previously described, and a second EPZ004777 molecule was bound in a pocket generated by yet a different conformation of the activation loop. The second EPZ004777 molecule did not appear in the structure obtained from SAH replacement, even when soaking at higher concentration of inhibitor. Taken together, these results indicate that the activation and substrate-binding loops are capable of adopting highly variable conformations from one crystal structure to another. Indeed, within the structured regions of the activation and substrate-binding loops, variability in atomic coordinates was evident also by crystallographic B-factors ( Fig. 4c–e ). 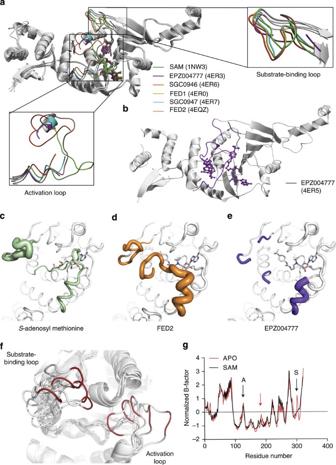Figure 4: Conformational variation of the DOT1L activation and substrate-binding loops. (a) The activation and substrate-binding loops adopt diverse conformations in complex with SAM (green),EPZ004777(magenta),SGC0946(orange),FED1(yellow),SGC0947(cyan) andFED2(beige). (b) Soaking of the 5-iodotubercidin-bound crystals withEPZ004777results in a complex that contains a second binding pocket occupied by a secondEPZ004777molecule. (c–e) Variability in atomic coordinates is evident in loop regions by crystallographic B-factors as illustrated by ribbon thickness in (c) SAM, (d)FED2and (e)EPZ004777complexes. (f) MD simulation of apo DOT1L (1NW3) shows a diverse population of loop conformations. (g) Quantification of protein flexibility through calculation of normalized MD B-factors identifies regions of high mobility in the activation loop (arrow labelled ‘A’) and substrate-binding loop (black arrow labelled ‘S’). SAM binding reduces MD B-factors near to the open SAM nucleoside-binding pocket. The PDB code of each structure is indicated. Figure 4: Conformational variation of the DOT1L activation and substrate-binding loops. ( a ) The activation and substrate-binding loops adopt diverse conformations in complex with SAM (green), EPZ004777 (magenta), SGC0946 (orange), FED1 (yellow), SGC0947 (cyan) and FED2 (beige). ( b ) Soaking of the 5-iodotubercidin-bound crystals with EPZ004777 results in a complex that contains a second binding pocket occupied by a second EPZ004777 molecule. ( c – e ) Variability in atomic coordinates is evident in loop regions by crystallographic B-factors as illustrated by ribbon thickness in ( c ) SAM, ( d ) FED2 and ( e ) EPZ004777 complexes. ( f ) MD simulation of apo DOT1L (1NW3) shows a diverse population of loop conformations. ( g ) Quantification of protein flexibility through calculation of normalized MD B-factors identifies regions of high mobility in the activation loop (arrow labelled ‘A’) and substrate-binding loop (black arrow labelled ‘S’). SAM binding reduces MD B-factors near to the open SAM nucleoside-binding pocket. The PDB code of each structure is indicated. Full size image In all structures, the crystal lattice is such that adjacent DOT1L molecules are in contact with both the activation and the substrate-binding loops. Thus, our observations of conformational heterogeneity of the loops and potential 2:1 binding stoichiometry derived from crystal structures might be influenced by surface contacts in the crystal lattice. We performed solution state binding studies in order to better understand these properties. SPR indicated unambiguously that the DOT1L:inhibitor complex has a binding stoichiometry of 1:1 for EPZ004777 and its four analogues ( Supplementary Fig. S5 ). This result was also confirmed by isothermal titration calorimetry for EPZ004777 ( Supplementary Fig. S6 ). The second inhibitor-binding site observed in one of our DOT1L– EPZ004777 complex structures is therefore most likely an artifact of the high concentration of inhibitor used for soaking, and/or crystal-packing contacts. Nevertheless, these structures clearly show that the substrate and activation loops of DOT1L are able to adopt a wide variety of conformations, suggesting a significant degree of flexibility and/or conformational mobility. Dynamical effects of inhibitors on the DOT1L catalytic site To explore the dynamic features of DOT1L, we performed 23 and 31 ns molecular dynamics (MD) production runs on DOT1L in the presence and absence of SAM, respectively. The initial coordinates were taken from crystallographic data and prepared as described in Supplementary Methods . For the dynamics of apo DOT1L, the coordinates of the cofactor were deleted from the protein–cofactor complex (PDB:1NW3). The system was stable (average RMS of 3.1 Å; Supplementary Fig. S7 ), and revealed a large conformational flexibility of the activation loop and substrate-binding loop as shown by the superposition of several snapshots saved along the MD ( Fig. 4f ) and quantified by the calculation of the theoretical B-factor per residue (computational approximations of the atomic displacement parameter; Fig. 4g ). The maximum flexibility is centred around residue W301 for the substrate-binding loop, and around residue P126 for the activation loop. A residue-by-residue comparison of molecular dynamical B-factors obtained from apo and SAM-bound simulations identified a putative region of conformational stabilization by engagement of the cofactor-binding site, spanning residues 183–193, which defines a portion of the substrate-binding pocket that engages the nucleoside features of SAM and analogous small-molecule inhibitors ( Fig. 4g ). These data support a model in which ligand binding partially organizes a highly flexible DOT1L catalytic site. With an interest in experimentally interrogating the conformational flexibility of DOT1L, we performed hydrogen exchange mass spectrometry (HX-MS) on apo DOT1L, as well as saturated complexes with selective small-molecule inhibitors and the cofactor product, SAH. With HX-MS, the relative dynamics within a protein are monitored by measuring the exchange of backbone amide hydrogens with the bulk solvent [24] . First, experimental methods were developed to provide adequate DOT1L catalytic domain protein coverage (>98%) following pepsin digestion ( Supplementary Fig. S8 ). We then sought to investigate if conformational or dynamic changes occur in DOT1L upon inhibitor binding and where the changes were located with respect to the substrate-binding site. Three inhibitors defining a broad range of target-specific biochemical inhibition for DOT1L were selected for study using HX-MS: SAH, FED2 and EPZ004777 . Hydrogen exchange was measured for each of the three inhibitors and the results were compared with the hydrogen exchange of DOT1L alone. As shown in Fig. 5a , apo DOT1L is a dynamic protein that exchanges amide hydrogens rather rapidly. Notably, rapid exchange was evident in both the substrate binding and activation loops at the earliest time point following deuterium exchange (10 s), indicating a relatively higher degree of solvent exposure and/or conformational flexibility consistent with crystallographic findings and computational predictions by MD. Exchange, and therefore dynamics, was comparable between apo DOT1L and DOT1L incubated with SAM-competitive inhibitors for the majority of the protein throughout the time frame of the experiment (1 h). However, certain regions demonstrated ligand-associated reduction in hydrogen exchange, consistent with meaningful changes in protein dynamics upon inhibitor binding. 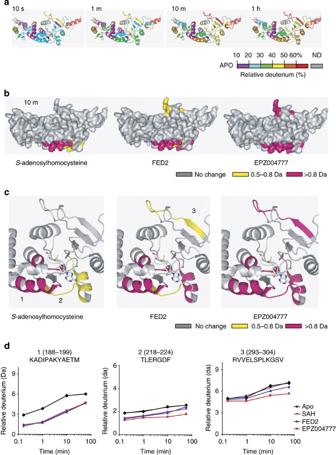Figure 5: Hydrogen–deuterium exchange. (a) Summary of all HX-MS data for DOT1L alone mapped onto the crystal structure of DOT1L. (b,c) Comparison of deuterium exchange with DOT1L inhibitor binding, as shown in a (b) space-filling model and (c) a ribbon model at higher magnification. The relative deuterium levels for all residues of DOT1L that were probed with hydrogen exchange are mapped with colour for each exchange point; the colour code is explained at the bottom of each figure. Regions coloured gray represent residues where deuterium levels were not determined (ND) or where there were no changes upon inhibitor binding. (d) The deuterium uptake curves for three representative peptides are shown. The maximum of theyaxis in each graph is the maximum amount of deuterium that could be incorporated. As these experiments were performed as comparisons under identical experimental conditions, no corrections have been made for back-exchange thus the absolute value of each deuterium level is 18–25% higher than plotted based on totally deuterated standards (described in detail in ref.24). The cumulative error of measuring deuterium uptake in these assays is ~±0.20 Da. Any differences larger than this value were considered significant for the purposes of comparing the datasets28. The location of each peptide, according to the labels, is shown on the crystal structures in (c). All HX-MS data are shown mapped to PDB:1NW3, for ease of comparison. Figure 5: Hydrogen–deuterium exchange. ( a ) Summary of all HX-MS data for DOT1L alone mapped onto the crystal structure of DOT1L. ( b,c ) Comparison of deuterium exchange with DOT1L inhibitor binding, as shown in a ( b ) space-filling model and ( c ) a ribbon model at higher magnification. The relative deuterium levels for all residues of DOT1L that were probed with hydrogen exchange are mapped with colour for each exchange point; the colour code is explained at the bottom of each figure. Regions coloured gray represent residues where deuterium levels were not determined (ND) or where there were no changes upon inhibitor binding. ( d ) The deuterium uptake curves for three representative peptides are shown. The maximum of the y axis in each graph is the maximum amount of deuterium that could be incorporated. As these experiments were performed as comparisons under identical experimental conditions, no corrections have been made for back-exchange thus the absolute value of each deuterium level is 18–25% higher than plotted based on totally deuterated standards (described in detail in ref. 24 ). The cumulative error of measuring deuterium uptake in these assays is ~±0.20 Da. Any differences larger than this value were considered significant for the purposes of comparing the datasets [28] . The location of each peptide, according to the labels, is shown on the crystal structures in ( c ). All HX-MS data are shown mapped to PDB:1NW3, for ease of comparison. Full size image Regional changes in HX-MS with ligand binding were observed most frequently near the cofactor-binding site, consistent with the mode of binding determined by crystallography ( Fig. 5b ). For example, all compounds contributed marked decreases in exchange in the region of peptide (188–199), consistent with structural and MD data that show improved conformational stability attributable to SAM nucleoside binding ( Fig. 5c ). Further stabilization of the interior face of the SAM-binding pocket was proportionate to inhibitor potency, evidenced by decreasing exchange in peptide (218–224) and peptide (160–172) in the presence of SAM, FED2 and EPZ004777 ( Fig. 5d , Supplementary Fig. S8 ). Upon binding by the potent DOT1L inhibitor EPZ004777 , considerably stronger effects on HX-MS were observed in peptide (293–304), which is precisely the structured region of the substrate-binding loop resolved by co-crystallographic studies as reorganized to accommodate the t-butylphenyl group ( Fig. 5c ). Taken together, our crystal structures, biochemical analysis and MD simulations indicate that the activation and substrate-binding loops of DOT1L are inherently flexible and that the cofactor and substrate-binding sites can undergo dramatic conformational remodelling to accommodate a variety of hydrophobic ligands. The DOT1L inhibitor structures presented here are the first structures of a PMT in complex with cofactor-competitive inhibitors that are active in cells. Integrated structural, biochemical, computational and biophysical analysis of DOT1L bound to a focused library of informative small-molecule inhibitors has defined a novel mode of inhibition, associated with active site remodelling and local stabilization of a highly dynamical protein target. The extensive and unexpected backbone motion induced by inhibitors may reflect a functional mechanism necessary for cofactor exchange following catalysis and enzymatic turnover. Based on the previous structural data of SAM-bound DOT1L [6] , the high-affinity, SAM-competitive binding of EPZ004777 [17] was puzzling for two reasons. First, EPZ004777 is a very hydrophobic compound, while the SAM pocket is hydrophilic. Second, it is significantly larger than SAM, and therefore would not be expected to fit into the SAM-binding pocket ( Fig. 2d ). Thus, binding of EPZ004777 to the cofactor site of DOT1L seemed to defy basic principles of shape and electrostatic complementarity. While the SAM-binding pocket of many PMTs is expected to be druggable [4] , the high polarity of the pocket represents a challenge for the design of small-molecule inhibitors sufficiently hydrophobic to cross cell membranes. EPZ004777 has emerged as an important first-generation selective inhibitor of DOT1L, exhibiting high target potency in cellular assays perhaps attributable to its hydrophobicity. However, this SAM analogue possesses limited solubility (50 μM in aqueous solution). Recently, additional mimetics of SAM were reported as nanomolar inhibitors of DOT1L, but no cellular activity was provided, perhaps owing to the high polarity of the compounds [20] , which would likely confer poor cellular permeability. Guided by crystallographic and computational data characterizing a focused library of DOT1L inhibitors, we observe remodelling of the catalytic site to accommodate bulky hydrophobic groups tethered by a urea linkage. As evidenced by the FED2 structure, for example, hydrophobic DOT1L inhibitors induce the formation of a largely enclosed binding pocket, which is on average 68% more hydrophobic than the corresponding site in all available structures of DOT1L in complex with SAM, SAH or close analogues ( Supplementary Fig. S9 ). The poor pharmacokinetic properties of EPZ004777 limit its utility as a chemical probe in the in vivo setting where much of the DOT1L developmental and disease biology is studied [10] , [11] , [25] . Indeed, in the article first reporting EPZ004777 , a pharmacological target validation study performed in a murine model of MLL required administration by osmotic pumps implanted subcutaneously to overcome evidently poor pharmacokinetics [17] . Our structural analysis clearly indicates positions of the compound that could be exploited to improve its pharmacokinetic properties and potency. Here, we show that SGC0946 has improved potency in cellular assays measuring the levels of H3K79 methylation. SGC0946 also has improved efficiency at specifically reducing the cell viability of a human MLL cell line derived from human cord blood that is transformed with the MLL-AF9 translocation oncogene [22] . SGC0946 specifically killed these MLL translocated cells but not cells transformed with another leukemogenic fusion protein [23] . Inhibition of histone methyltransferases is a promising new avenue for therapeutic discovery [1] , [3] , and potent, selective and cell permeable reagents are urgently needed to link pharmacological inhibition of specific PMTs with desirable phenotypes. We show here that remodelling of the DOT1L cofactor pocket allows competition by chemical inhibitors with physico-chemical properties distinct from and more drug-like than those of SAM. We suggest that this phenomenon may be a general principle that could be exploited for other PMTs. Indeed, the Post-SET element of SET-domain methyltransferases, and the α-X helix of PRMTs, both located at the SAM-binding site, are flexible and dynamic regions that adopt a catalytically competent conformation upon SAM binding [26] , [27] . The potent DOT1L inhibitor SGC0946 demonstrates how limited chemical modification can significantly improve cellular activity, probably a direct effect of a lower K D , extended residence time and improved permeability [21] . Importantly, this compound (available from the Structural Genomics Consortium for research purposes) will serve as a useful chemical probe [19] to further investigate the cellular mechanism of DOT1L in both normal and diseased cells. Furthermore, structural resolution of the mode of molecular recognition of DOT1L by prototype inhibitors using data and methods outlined here will guide development of improved compounds and will accelerate the development of clinical candidates. Crystallization Protein expression and purification are described in Supplementary Methods . To obtain crystals of DOT1L(1-351)/ EPZ004777 , crystals of DOT1L(1-351) with SAH were first prepared for displacement soaking. Crystals of DOT1L (1–351) complexed with SAH were obtained at 18 °C using the vapour diffusion method by mixing a protein solution at a concentration of 20 mg ml −1 (in 20 mM Tris–HCl pH 8.0, 200 mM NaCl, 1 mM EDTA and 1 mM tris(2-carboxyethyl)phosphine) with a fivefold excess of SAH with an equal volume of reservoir solution (1.6 M (NH 4 ) 2 SO 4 , 0.01 M MgCl 2 , 0.1 M Na Cacodylate, pH 5.5). Solid EPZ004777 was dissolved in Milli-Q water to obtain a 10 mM stock solution. For soaking, 1 μl of 10-mM EPZ004777 stock solution was mixed with 19 μl of reservoir buffer to prepare 0.5 mM EPZ004777 in soaking buffer. Crystals of DOT1L(1-351)/SAH were transferred into 1.5 μl soaking buffer and incubated for 12 h during which time EPZ004777 displaced SAH in the crystals. To obtain crystals of DOT1L (1–420) with FED1 , FED2 , SGC0946 , SGC0947 and EPZ004777 , crystals of DOT1L(1–420)/5-iodotubercidin were first prepared for displacement soaking. Purified protein DOT1L (1–420) was concentrated to 16 mg ml −1 in a buffer containing 20 mM Tris–HCl pH 8.0, 200 mM NaCl, 1 mM EDTA and 1 mM tris(2-carboxyethyl)phosphine. To obtain crystals of DOT1L/5-iodotubercidin, DOT1L (1–420) was mixed with 5-iodotubercidin by directly adding a fivefold molar excess of compound to the protein solution, and the sitting drop vapour diffusion method was used at 18 °C in a buffer containing 3.5 M sodium formate, and 100 mM sodium acetate, pH 4.6. For displacement soaking, all solid compounds were first dissolved in Milli-Q water to obtain 10-mM aqueous stock solutions. Compound solutions for displacement soaking were prepared by diluting 1 μl stock solution of each compound with 19 μl reservoir buffer to make 0.5 mM compound solutions. Crystals of DOT1L (1–420)/5-iodotubercidin were then transferred into 1.5 μl of each compound solution and incubated for 4–24 h at 18 °C. Before being flash-frozen in liquid nitrogen, the crystals were soaked in a cryoprotectant consisting of 80% reservoir solution and 20% glycerol. DOT1L methyltransferase assay The reported assay condition was used with minor modification [17] . Nucleosomes purified from chicken blood cells was used as substrate. Sixty nanomolar nucleosome solution was added into 40 μl assay buffer (20 mM Tris–HCl, 2 mM DTT, 10 mM MgCl 2 and 0.01% Triton X-100), which contained 0.25 nM recombinant DOT1L (1–420) with inhibitors of different concentrations (or dimethylsulphoxide (DMSO) as control). A similar 40 μl mixture without DOT1L was prepared as background. The mixture was incubated at room temperature for 30 min before 0.75 μM 3H-SAM (PerkinElmer, catalogue number NET155001MC) was added to start the reaction. The reaction mixture was incubated at room temperature for 2 h and quenched by the addition of 160 μl 10% trichloroacetic acid. The mixture was transferred into glass fibre filter plates (Millipore, catalogue number MSFBN6B) and washed twice with 10% trichloroacetic acid. An ethanol wash (100 μl) was followed by drying. One hundred microlitre Microscint Zero (PerkinElmer, catalogue number 6013611) was finally added into each well of the filter plates and centrifuged to flow through filters. Tritium incorporation was detected on a TopCount (PerkinElmer). Inhibitor selectivity profiling Selectivity of DOT1L inhibitors was assessed by screening a panel of SAM-dependent methyltransferases (SUV39H2, G9a, EHMT1, SETDB1, PRMT3, SETD7, MLL, SETD8, SUV420H1, SUV420H2, PRC2, DNMT1 and PRMT5) by a radioactivity-based assay (conditions in Supplementary Table S4 ). In this assay, 3H-SAM (Cat.# NET155V250UC, Perkin Elmer) was used as a methyl donor to methylate peptide substrates. Peptide substrates were biotinylated to be captured in each well through their interaction with streptavidin using a streptavidin-coated flash plate (96-well FlashPlate, Cat#: SMP103, Perkin Elmer, http://www.perkinelmer.com/ ). Amount of the product (methylated peptide) was quantified by tracing the radioactivity (counts per minute measured by a TopCount reader from Perkin Elmer). Assay conditions were optimized for each protein separately, and all experiments were performed at linear initial velocity. The enzymatic reactions were conducted in triplicate at room temperature for 1 h in a 20 μl reaction mixture in 20 mM Tris–HCl, pH 8.0, 5 mM DTT and 0.01% Triton X-100 containing 3H-SAM at concentrations around or below the Km value of each enzyme. The reaction was quenched with equal volumes of 7.5 M guanidine-HCl. Ten microlitres of the reaction mix containing guanidine-HCl was mixed with 190 μl of 20 mM Tris Buffer, pH 8 and transferred into a flash plate. The plate was incubated for an hour before reading using a TopCount (Perkin Elmer, http://www.perkinelmer.com/ ) to accumulate maximum signal. Surface plasmon resonance SPR studies were performed using a Biacore™ T200 instrument (GE Health Sciences Inc.). DOT1L (1–420, ~4000RU) was stably immobilized to CM5 chips through amine coupling at pH 7.4 according to the manufacture’s protocol (GE Health Sciences Inc.). Compounds were dissolved in 100% DMSO and twofold serial dilutions were performed in 100% DMSO. For testing, the serially diluted compounds were diluted 1:20 into HBS-EP buffer (20 mM HEPES pH 7.4, 150 mM NaCl, 3 mM EDTA and 0.05% P-20) giving a final concentration of 5% DMSO. The flow rate was set at 70 μl min −1 . For each compound, single-cycle kinetic analysis was performed with an on-time of 300 s, and an off-time of 1800, s. SAM and SAH were used as positive controls. Curve fitting and K D determinations were performed with the Biacore T200 Evalutation software (GE Health Sciences Inc.). Five concentrations of each compound were tested in twofold serial dilution experiments within the ranges listed. All compounds were fitted using the on and off rates, which were then used to calculate the K D . The stoichiometry was determined by reference to the binding levels of the 1:1 binding controls, SAM and SAH. The SPR profile is unusual for the most potent compounds owing to their extreme binding affinity. The results were based on four independent repeats. Immunoblot of H3K79me2 For western blot analysis in human cell lines, exponentially growing human leukaemia cell line MV4;11 or Molm13 cells were plated in 6-well plates at 2 × 10 5 cells per well in a final volume of 2 ml. Cells were incubated in the presence of DMSO or 10 μM of EPZ004777 or other synthesized derivatives, excepting SGC0946 that was incubated at a concentration of 1 μM. For the Molm13 experiments, 1 μM of compounds were used for times indicated. Cells (2–4 × 10 6 ) were harvested at 4 days (MV4:1) and histones were extracted as detailed in Methods. Histones (3 μg) were separated on 10% Bis-Tris gels (Invitrogen NP0315BOX), transferred to 0.2 μM nitrocellulose membranes using the IBLOT and probed with the appropriate primary antibodies diluted 1:1000 in 5% milk in TBS-T. Following primary antibody incubation, membranes were probed with ECL donkey anti Rabbit IgG (Thermo Fisher Scientific 45-000-683) secondary antibody and signal was detected using SuperSignal West Pico Chemiluminescent Substrate Fisher Scientific (Thermo Fisher Scientific PI-34077). Cellular H3K79 methylation assay MCF10A cells were grown in DMEM/F12 5% horse serum, EGF (20 ng ml −1 ), hydrocortisone (0.5 μg ml −1 ), cholera toxin (100 ng ml −1 ) and insulin (10 μg ml −1 ) in 96-well plates in the presence of inhibitors as stated in figures. Media were removed by flicking and 200 μl of 0.3%Triton, 0.1% SDS and 2% formaldehyde in PBS for 10 min. After five washes with 0.1% Triton X100 in PBS, cells were blocked for 1 h with 200 μl of blocking buffer (0.5% Triton, 3% BSA and 5% goat serum azide PBS) with 0.25 M glycine. Three replicate wells for each concentration were exposed to H3K79m2 antibody (Abcam Ab3594) in the blocking buffer with 0.1% SDS at 1:1000 dilution overnight. The wells were washed five times with 0.1% Tween 20 in PBS, then incubated with secondary IR800 conjugated antibody (LiCor 926-32211) and DNA-intercalating dye, DRAQ5 (LiCor) for 1 h. After five washes with 0.1% Tween 20 PBS, the plates were read on an Odyssey scanner (LiCor) at 800 nm (H3K79m2 signal) and 700 nm (DRAQ5 signal). Fluorescence intensity was quantified, normalized to background and DRAQ5 signal, and expressed as a percentage of control. Cell viability Human cord blood cells transformed with MLL-AF9 or TLS-ERG were cultured as described elsewhere [22] , [23] . The cells were treated with DMSO or inhibitor at 1 and 5 μM for 14 days. Cell viability assay was performed by incubating cells with resazurin solution (0.1 mg ml −1 ) for 4 h and fluorescent resorufin measurement at 584 nM. Gene expression assay RNA was extracted using Qiazol reagent, reverse transcribed (qScript, Quanta Biosciences) according to the manufacturer’s instructions and PCRs performed with iTaq SYBR green reagent (BioRad) using primers: HOXA9 5′-TGCTGAGAATGAGAGCGGCGGA-3′ and 5′-GCACCGCTTTTTCC GAGTGGA-3′, Meis1 5′-CCCCCGCTGCTGTCTTGGAAAC-3′ and 5′-CCTACTCCATCCATGCCCCCGT-3′. The data were normalized to the TBP endogenous control. Accession codes: The coordinates and structure factors for human DOT1L complex structures presented in this work have been deposited in the Protein Data Bank (PDB) with the following accession numbers: single EPZ004777 molecule: 4ER3 ; 5-iodotubercidin: 3UWP ; SGC0946 : 4ER6 ; FED1 : 4ER0 ; SGC0947 : 4ER7 ; FED2 : 4EQZ ; two EPZ004777 molecules: 4ER5 . How to cite this article: Yu, W. et al . Catalytic site remodeling of the DOT1L methyltransferase by selective inhibitors. Nat. Commun. 3:1288 doi: 10.1038/ncomms2281 (2012).